The function of zebra stripes Despite over a century of interest, the function of zebra stripes has never been examined systematically. Here we match variation in striping of equid species and subspecies to geographic range overlap of environmental variables in multifactor models controlling for phylogeny to simultaneously test the five major explanations for this infamous colouration. For subspecies, there are significant associations between our proxy for tabanid biting fly annoyance and most striping measures (facial and neck stripe number, flank and rump striping, leg stripe intensity and shadow striping), and between belly stripe number and tsetse fly distribution, several of which are replicated at the species level. Conversely, there is no consistent support for camouflage, predator avoidance, heat management or social interaction hypotheses. Susceptibility to ectoparasite attack is discussed in relation to short coat hair, disease transmission and blood loss. A solution to the riddle of zebra stripes, discussed by Wallace and Darwin, is at hand. The striking black and white striped pelage of zebras has intrigued people for millennia and has captured the attention of many biologists [1] , [2] , [3] , [4] but its adaptive significance remains unsolved. Functional hypotheses fall into five broad categories: a form of crypsis probably matching a woodland background, disrupting predatory attack, reducing thermal load, having a social function and avoiding ectoparasite attack [5] , [6] , [7] . Only two have received more than passing attention: humans find moving striped objects difficult to target accurately on a computer screen, suggesting a possible motion dazzle confusion effect [8] , [9] , [10] , and tsetse flies, stomoxys stable flies and tabanid biting flies are less likely to land on black and white striped than on uniform surfaces [11] , [12] , [13] , [14] . Of the seven extant wild equid species, three have prominent black and white stripes (plains, Equus burchelli ; mountain, E. zebra ; and Grevy’s zebra, E. grevyii ), whereas the grey African wild ass ( E. africanus ) has thin stripes on its lower legs. The three Asiatic species (Kiang, E. kiang , Asiatic wild ass, E. hemionus and Przewalski’s horse, E. ferus przewalskii ) have no stripes but have grey or brown coats that undergo moult in parts of their ranges. Equid subspecies show considerable variation in striping pattern too [15] . We capitalized on this variation by matching species’ and subspecies’ geographic range overlaps to factors proposed for driving the evolution of zebras’ extraordinary coat colouration. While conspecific with E. ferus przewalskii , we excluded domestic and feral horses because their coat colour is labile and has been subject to intense selection through domestication [16] . Controlling for phylogeny both at the subspecies level as well as at the species level, we test (i) whether black and white stripes are a form of crypsis, matching the background of light and dark produced by tree trunks and branches in woodland habitats [4] . To investigate an antipredator function that subsumes several mechanisms including crypsis [3] , disruptive colouration of the body’s outline [17] , increased apparent size [18] , making individuals difficult to single out in a herd [19] , confusing a predator in some way [6] , [9] or advertising flight ability [20] , we examine (ii) whether striping in equids is associated with the presence of sympatric large predators: spotted hyaena ( Crocuta crocuta ), lion ( Panthera leo ), tiger ( P. tigris ) and wolf ( Canis lupus ). (iii) To explore heat management [6] , we examine associations between striping and living in habitats with average maximum annual temperatures of 25 °C through to 30 °C. (iv) We use average group size and maximum herd size as coarse indicators of the involvement of striping in social interactions [6] , [21] . To investigate the importance of biting flies [22] , [23] , we match (v) tsetse fly distributions to equid distributions and use environmental proxies for the distribution of tabanid abundance. Overall striping In just single-factor analyses at the species level (see Methods), the presence of body stripes was very strongly associated with presence of tsetse flies, with several measures of tabanid fly activity and with presence of lions. For geographic distributions of tsetse flies, for between 5 and 11 consecutive months of good conditions for tabanids, and for the presence of lions, the striped equid species with the lowest geographic range overlap on each of these measures still had greater percentage overlaps than the highest percentage overlap scores of non-striped species. In these cases of a ‘perfect’ fit (that is, separation), the maximum likelihood estimate does not exist, so traditional logistic regression and phylogenetically corrected tests are impossible [24] . In contrast, we found no significant associations of presence of body stripes with spotted hyaenas (phylogenetic logistic regression: N =7; P =0.403), woodland ( P =0.788) or any maximum temperature from 25 to 30 °C ( P =0.432–0.803), mean ( P =0.951) or maximum group sizes ( P =0.956) in single-factor analyses controlling for phylogeny. At the subspecies level, body stripe presence ( E. burchelli quagga scored as yes) was again ‘perfectly’ associated with the presence of tsetse fly distribution such that we could not run the statistical test. In contrast, we found no significant associations with 7 consecutive months of tabanid activity (phylogenetic logistic regression: N =20; P =0.4347), hyaena ( P =0.818), woodland ( P =0.9257) or lion ( P =0.9555) distributions, any maximum temperature ( P =0.5849–0.7447), mean ( P =0.7724) or maximum group sizes ( P =0.5998) in single-factor analyses. Striping on different parts of the body We next examined different parts of the body separately because striping may be found only in certain areas (for example, legs and body of E. africanus and fore and hindquarters of the extinct E. b. quagga ). 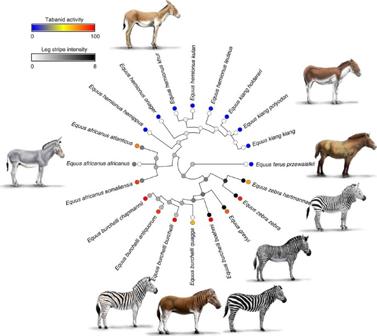Figure 1: Striping and tabanid activity. Phylogenetic tree of equid subspecies showing leg stripe intensity (inside circles) and proportion of geographic range overlap with 7 consecutive months of temperature lying between 15 and 30 °C and humidity between 30 and 85% (outside circles). Drawings by Rickesh Patel. (a) The number of face stripes was associated with 6 months of consecutive tabanid activity at the subspecies level (phylogenetic generalized least squares (PGLS): Z=2.522, N =20 P =0.012, I =0.87; Table 1A ) and marginally associated with 9 months of consecutive tabanid activity at the species level (PGLS: Z =1.938, N =7, P =0.0526, I =0.29; Table 1B ). (b) The number of neck stripes was associated with 6 months of consecutive tabanid activity (PGLS: Z =1.961, N =20, P =0.05, I =0.67; Table 1A ) at the subspecies level and marginally with 9 months of activity at the species level (PGLS: Z =1.909, N =7, P =0.0563, I =0.28; Table 1B ). (c) Flank striping was strongly associated with 8 months of tabanid activity at the subspecies level (PGLS: Z =2.209, N =20, P =0.0272, I =0.77; Table 1A ) with no factor significant at the species level ( Table 1B ). (d) At the subspecies level, rump striping was significantly associated with 9 months of tabanid activity (PGLS: Z =1.974, N =20, P =0.0484, I =0.67) and marginally with tsetse distribution (PGLS: Z =1.859, N =20, P =0.0630, I =0.60; Table 1A ). At the species level, rump striping was significantly associated with hyaena distribution (PGLS: Z =2.592, N =7, P =0.0095, I =0.60; Table 1B ). (e) Severity of shadow striping was strongly associated with 6 months of tabanid activity at the subspecies level (PGLS: Z =2.515, N =20, P =0.0119, I =0.87; Table 1A ) but we were unable to run a multifactorial logistic regression at the species level because shadow stripes are only found in the plains zebra, although this species does have the highest tabanid activity score of any equid (that is, presence of shadow stripes is ‘perfectly’ associated with tabanid activity). (f) Belly stripe number was strongly associated with tsetse fly distribution at the subspecies level (PGLS: Z =5.034, N =20, P =5 × 10 −7 , I =1.00; Table 1A ). At the species level, it was strongly associated with tsetse fly distribution (PGLS: Z =2.862, N =7, P =0.0042, I =0.66) and marginally with woodland (PGLS: Z =1.815, N =7, P =0.0695, I =0.11; Table 1B ). (g) Leg stripe density was significantly associated with 7 months of tabanid activity (PGLS: Z =2.726, N =20, P =0.006, I =0.87; Table 1A ) at the subspecies level ( Fig. 1 ). Leg stripe density was associated with lion distribution (PGLS: Z =2.195, N =7, P =0.0282, I =0.36) and marginally with 7 months of tabanid activity at the species level (PGLS: Z =1.820, N =7, P =0.0687, I =0.19; Table 1B ). Table 1 Full phylogenetic generalized least squares models showing associations between measures of striping and environmental factors. Full size table Figure 1: Striping and tabanid activity. Phylogenetic tree of equid subspecies showing leg stripe intensity (inside circles) and proportion of geographic range overlap with 7 consecutive months of temperature lying between 15 and 30 °C and humidity between 30 and 85% (outside circles). Drawings by Rickesh Patel. Full size image There are many hypotheses for striping in zebras: (i) camouflage against predators through (a) background matching or (b) disruptive colouration; (ii) avoiding being killed by predators through confusion by (a) misjudging the number of zebras in the group, (b) the size of the target, (c) flight speed, or through (d) quality advertisement or (e) aposematism; (iii) cooling the animal; (iv) social factors, namely, (a) individual recognition, (b) social stimulation of conspecifics, (c) causing individuals to group together, (d) directing grooming at certain parts of the body or (e) mate choice; and (v) avoidance of biting flies, be they (a) glossinids or (b) tabanids. Our comparative analyses that pit the five principal hypotheses against each other indicate that biting flies (hypotheses v(a) and v(b)) are the evolutionary drivers for striping in equids, at least on most regions of the body ( Table 1 ). Many of our independent variables were highly intercorrelated; for instance, spotted hyaenas inhabit the hot tropics and subtropics [25] and tsetse flies rest on trees [26] . Therefore, we can only be confident of our findings stemming from a model selection procedure that pits factors against each other to see the relative importance of each in explaining variation across all possible models. Regarding the possible effect of biting flies as evolutionary drivers for striping in equids, our significant findings were (i) that presence of body stripes is associated with tsetse fly distribution and between 5 and 11 consecutive months of tabanid activity at the species level, and with tsetse fly distribution at the subspecies level; (ii) that aspects of face, neck, flank, rump striping and shadow stripes are associated with between 6 and 9 consecutive months of tabanid activity at the subspecies level; and (iii) and that belly stripe number is associated with tsetse fly distribution at the subspecies level and with tsetse flies and marginally with woodlands at the species level. Indeed, the ranges where tabanids and tsetse flies are active matches that of striped equids well ( Fig. 2 ). We had estimated 15–30 °C and 30–85% humidity as ideal conditions for tabanid activity and reproduction (see Methods) but recognize that Culicidae (mosquitoes), Stomoxys (Muscidae, stable flies) and Simuliidae (blackflies) are abundant in the wet season too [27] . While the association between striping and warm humid months might imply stripes being a means of reducing heat load, this seems unlikely, given the lack of association with any maximum temperature in any multivariate model. 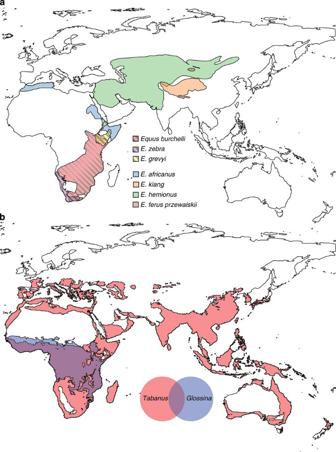Figure 2: Distributions of equids, tabanids and glossinids. (a) Map of the Old World showing distribution of 7 species of equids. (b) Distribution of tsetse flies (Glossina) and location of 7 consecutive months of tabanid activity (see methods). Figure 2: Distributions of equids, tabanids and glossinids. ( a ) Map of the Old World showing distribution of 7 species of equids. ( b ) Distribution of tsetse flies (Glossina) and location of 7 consecutive months of tabanid activity (see methods). Full size image Instead, our results lend strong ecological and comparative support to experiments that show that some tsetse and tabanid species avoid black and white striped surfaces [11] , [12] , [13] , [14] . Biting flies are attracted to hosts by odour, temperature, vision and movement that may act at different stages during host seeking, but vision is thought to be important in the landing response [27] with dark colours being particularly attractive [28] . Waage [11] found that black and white striped models caught fewer Glossina morsitans and G. pallidipes in the field than black or white models whether moving or stationary, and similar results were found for tabanids. He argued that stripes might obliterate the stimulus of the body edge or reduce the amount of contrast of the animal’s form against its background or be too narrow to elicit attraction. He believed that attraction from a distance rather than the landing response was affected by striping. Brady and Shereni [13] found similar results for G. morsitans and Stomoxys calcitrans demonstrating reduced landings as stripe number and thinness increased. Gibson [12] showed that horizontal stripes of 5 cm were actually avoided by tsetse and that vertical stripes were much less attractive than black or white surfaces (although similar to grey). She suggested that horizontal stripes might appear to a tsetse fly to be inconspicuous patches of dark and light, while the edges of the animal perpendicular to the alignment of stripes might be difficult to detect because of the absence of lateral inhibition. It is therefore noteworthy that stripes on all parts of the body except the forehead lie perpendicular to the outline of the zebra’s body. Egri et al . [14] showed that tabanids are less likely to land on black and white striped surfaces than uniform black or (arguably) white surfaces, that this effect is more marked as stripe width declines and that the most effective deterrent stripe widths used in their experiments matched the range of stripe widths found on the three species of zebra. From the literature, we recalculated glossinid, tabanid and stomoxys preferences for varying stripe widths. Zebra stripe widths on most parts of the body fall in a range lower than those preferred by all three groups of biting flies ( Fig. 3 ) extending the analysis by Egri et al . [14] to two other families of biting flies. It is noteworthy that stripes nearer the ground (on the legs and head when grazing) are especially thin and biting flies prefer to alight on shaded parts of animals low on the body [28] . Specifically, tabanids cruise at around 30 cm above ground and prefer alighting on lower legs of cows [29] , although the particular area differs by species; stable flies concentrate low on cows’ bodies as do blackflies, and tsetse flies prefer to feed on the hocks of cattle [30] . Interestingly, faint leg striping is sometimes seen on some Przewalski’s horse individuals, although on none in our sample. 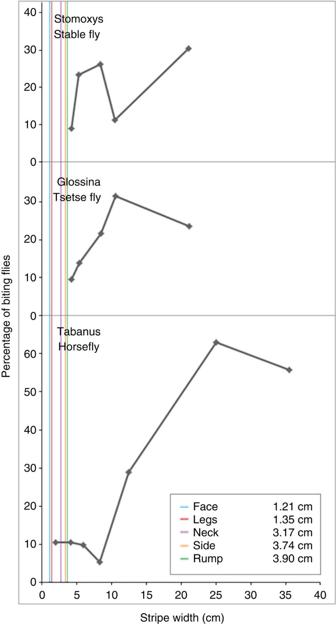Figure 3: Biting fly preferences and stripe widths. Percent of biting flies landing on stripes of varying widths. Stomoxys and Glossina from ref13, Tabanidae from ref14. Vertical lines show average stripe widths taken from (left to right) face, legs, neck, flank and rump averaged across the three species of zebra. Figure 3: Biting fly preferences and stripe widths. Percent of biting flies landing on stripes of varying widths. Stomoxys and Glossina from ref 13 , Tabanidae from ref 14 . Vertical lines show average stripe widths taken from (left to right) face, legs, neck, flank and rump averaged across the three species of zebra. Full size image Is there evidence that zebra striping deters biting flies from landing? Indirect observations are suggestive. First, incidence of tsetse blood meals derived from zebras is low [31] particularly in G. morsitans . Second, the incidence of trypanosomiasis carried by tsetse flies is either comparable to sympatric mammals or lower [32] , whereas domestic horses (unstriped) suffer badly from this disease in many parts of Africa [33] . Elsewhere, feral and semidomesticated horses can be plagued by flies [34] . Many herbivores and feral horses are subject to intense fly annoyance that can reduce time spent feeding, and ameliorate attack by moving to different habitats [35] , resting [36] , retreating to shade [37] or grouping together [38] . Why, therefore, should African equids be so sensitive to biting flies and have evolved morphological as well as behavioural defenses? At a proximal level, hair depths and lengths of zebras are shorter than sympatric African artiodactyls and Przewalski’s horse ( Fig. 4 ) either potentially making them more susceptible to biting flies probing perpendicularly or burrowing into and against the hair shafts, or that stripes are a sufficient deterrent to allow zebras to have cropped pelage. Moreover, unlike Asiatic equids, zebras do not have thick winter coats. Biting fly mouthpart lengths are markedly longer than average hair depths of zebras and approximately the same as zebra hair lengths ( Fig. 4 ), perhaps making zebras particularly susceptible to annoyance. 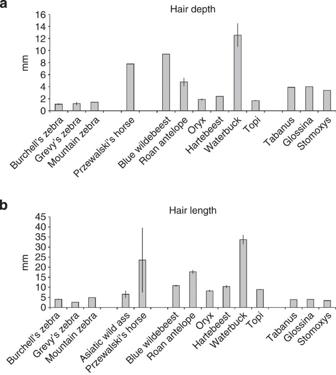Figure 4: Pelage characteristics of herbivores. Mean and s.e. hair depths (above) and mean and s.e. longest hair lengths (below) of zebra species, non-striped equids and artiodactyls living sympatrically with zebras measured using standard techniques.E. burchelli(5, 14 pelts, respectively)E. grevyi(3, 6),E. zebra(1, 1),E. hemionus(0, 7),E. ferus przewalskii(1, 2), blue wildebeestConnochaetes taurinus(1, 8), roan antelopeHippotragus equinus(4, 18), OryxOryx gazella(3, 9), hartebeestAlcelaphus buselaphus(1, 7), waterbuckKobus ellipsiprymnus(3, 9) and topiDamaliscus lunatus(7, 13). Lengths and depths calculated from taking the averages of at 7 points on the body (neck, flank, belly, rump, upper and lower foreleg and hindleg) for each pelt and averaging across pelts. Also shown are lengths of mouthparts of biting flies. Figure 4: Pelage characteristics of herbivores. Mean and s.e. hair depths (above) and mean and s.e. longest hair lengths (below) of zebra species, non-striped equids and artiodactyls living sympatrically with zebras measured using standard techniques. E. burchelli (5, 14 pelts, respectively) E. grevyi (3, 6), E. zebra (1, 1), E. hemionus (0, 7), E. ferus przewalskii (1, 2), blue wildebeest Connochaetes taurinus (1, 8), roan antelope Hippotragus equinus (4, 18), Oryx Oryx gazella (3, 9), hartebeest Alcelaphus buselaphus (1, 7), waterbuck Kobus ellipsiprymnus (3, 9) and topi Damaliscus lunatus (7, 13). Lengths and depths calculated from taking the averages of at 7 points on the body (neck, flank, belly, rump, upper and lower foreleg and hindleg) for each pelt and averaging across pelts. Also shown are lengths of mouthparts of biting flies. Full size image At an ultimate level, blood loss from biting flies can be considerable. Calculations show that blood loss from tabanids alone can reach 200–500 cc per cow per day in the United States [39] . For example, in Pennsylvania, mean weight gain per cow was 37.2 lbs lower over an 8-week period in the absence of insecticide that prevented horn fly ( Siphona ), stable fly ( Stomoxys ) and horse fly ( Tabanus ) attack [40] , and in New Jersey, milk production increased by 35.5 lbs over a 5-week period with insecticide [41] . Milk loss to stable flies was calculated at 139 kg per cow per annum in the United States [42] . Similarly, blood-sucking insects have been shown to negatively affect performance in draft horses [43] . Alternatively or additionally, striped equids might be particularly susceptible to certain diseases that are carried by fly vectors in sub-Saharan Africa [44] . We collated literature on diseases carried by biting flies that attack equids in Africa ( Supplementary Table 1 ) and note that equine influenza, African horse sickness, equine infectious anaemia, and trypanosomiasis and are restricted to equids, all are fatal and all are carried by tabanids. Currently, we are unable to distinguish whether zebras are particularly vulnerable or susceptible to biting flies because they carry dangerous diseases or because of excessive blood loss, but we are inclined towards the former because Eurasian equids are not striped, yet demonstrably subject to biting fly annoyance [37] . Background matching, heat management, facilitation of social interactions and predation have been also suggested as evolutionary drivers for striping in equids. Regarding background matching, we found no evidence for stripes being associated with woodland habitats, a lack of support for background matching against large mammalian predators in this environment. For subspecies, there was a marginal association between number of belly stripes and living in woodland habitat, but we suspect this derives from the close association between tsetse flies and woodlands rather than striping being a form of crypsis. Indeed, we found no evidence of striping elsewhere on the body being associated with woodland habitat, and it is difficult to envisage belly striping as a form of background matching, given its ventral position. Many artiodactyls have light or white stripes and spots set on a light or dark brown background that differ greatly from the sharp high contrast markings on zebras. Adult artiodactyls that have striped coats live in lightly wooded forests and those with striped young hide their offspring at birth [45] . Equids, on the other hand, are an open country clade with asses inhabiting deserts, zebras inhabiting tropical grasslands and horses living in temperate grasslands. Striped equids spend much of their time in open habitats and their foals follow their mothers from birth, which, respectively, demote the importance of striping being a form of background matching against trees and being a form of crypsis for young; background matching against grassland has been discounted by other authors [46] . Heat management does not appear as a driver for equid stripes either. There were no significant associations between striping at species or subspecies levels and inhabiting hot areas using six maximum temperature measurements. In fact, all equids live in open areas and temperatures can be very high in parts of the geographic range inhabited by E. burchelli and E. grevyi (east and southern Africa, northeast Africa, respectively) and unstriped E. africanus and E. hemionus (northeast Africa and central southern Asia, respectively) and both striped and unstriped equids manage heat stress by seeking shade if available. While black and white stripes might set up convection currents, E. zebra and E. burchelli often have thick black stripes running transversely along the dorsum, which would absorb heat especially when the sun is overhead. A social function cannot explain striping in equids either. We found no significant associations between striping and group size measures, although we acknowledge that these are coarse measures of the relative intensity of social interactions that unfortunately have received uneven attention across equid species. Generally, equids have two sorts of social system: a single stallion that lives with a small harem of mares and non-harem holding stallions that form small bands. This (type I) system [47] is characteristic of E. zebra , E. burchelli and E. przewalskii . The type II system ( E. grevyi , E. africanus , E. kiang and E. hemionus ) consists of loose bands of animals that collect together in medium sized to large aggregations at certain times of the year, long-lasting associations only occurring between mare and foal. Here individual recognition based on stripe pattern might be advantageous but three out of these four species do not have body stripes. Given that domestic horses are capable of recognizing other individuals [48] using visual, auditory and olfactory cues [49] , it seems unlikely that stripes are a critical means of identification. Predation has been the predominant factor included in a number of hypotheses for body striping in equids centering on avoiding predation through confusing predators, tricking them into misjudging the size of their prey or the speed of the prey, thereby miscalculating the final leap, by making it difficult to single out a member of the herd or through aspects of striping being a signal of individual quality tied to flight speed [10] , [19] , [21] , [50] , [51] . All indicate that stripes should have evolved in the presence of large predators, yet there was no strong congruence between striping on any part of the animal at the species or subspecies level and close sympatry with lions, except for leg stripe intensity at the species level, driven particularly by the extinct Barbary lion and extinct Altas African wild ass co-occurring in the Maghreb. Across contemporary ecosystems in Africa, where lions have been subjects of repeated detailed study, lions capture zebra in significantly greater proportions to their abundance [52] , suggesting that stripes are not an antipredator defence against lions acting through confusion, dazzle or other means. Despite the popularity of various sorts of confusion hypotheses, our data provide little support for this idea. In contrast, spotted hyaenas, a smaller predator than lions, capture fewer zebras than predicted by their relative abundance [53] . Hyaenas find it difficult to pull down an adult zebra because zebras deliver sharp kicks and bites to these predators; instead, hyaenas concentrate mostly on foals [25] . We found significant associations between rump striping and leg stripe intensity at the species level, so the possibility that striping in these areas of the body (where coursing predators might have prolonged views) is an aposematic signal to warn spotted hyaenas (and perhaps leopards P. pardalis and cheetahs Acinonyx jubatus ) to keep away cannot be dismissed entirely. Nonetheless, there were no significant species associations between hyaena distribution and striping measures on other areas of the body, and none at the subspecific level: aposematic deterrence of hyaenas may be a secondary benefit of stripes but cannot explain the presence of stripes on zebras more generally. In parts of Asia once inhabited by tigers and wolves, equids are not striped. These analyses tease apart long-standing but mainly untested hypotheses for the functions of striping in equids and lend strong ecological support for striping being an adaptation to avoid biting flies. Nonetheless, caution is warranted. First, our attempts to extract variables to test each hypothesis are inexact: plotting the distribution of tabanids was very difficult as there are no range maps for the >4,000 species and estimates of abundance are restricted to isolated study sites often in the New World. We hope that future studies can generate better quantitative spatial measures of tabanid annoyance. However, we are confident about historical tsetse fly distributions, historical predator ranges and annual temperatures. A second issue is that the sample size available with which to test hypotheses for striping in equids is small because there are only 7 extant species and 23 subspecies for which we have coarse environmental information, 3 of the latter had to be dropped owing to inadequate resolution of our phylogenetic tree. Furthermore, tree reconstruction at the species level shows that striping evolved only once in this clade. These caveats notwithstanding, it is reassuring that the sequence of studies indicating that biting flies shun striped surfaces, first put forward by Harris [22] in 1930, has been given ecological validity by our finding that striping on equids is perfectly associated with increased presence of biting flies. Stripes and background colouration To measure equid pelage colouration, we analysed coat patterns and colours using images of extant and extinct equid subspecies obtained from reputable sources online and in print ( Supplementary Note 2 ). Only 1 animal per photograph was scored, and we scored a maximum of 12 animals per subspecies (see Supplementary Note 2 for Ns). Images were only scored if the animal was identified with the proper scientific and common name, and if the location where the image was shot was identified to occur within the species’ (or subspecies’) known range. In total, we scored the following seven species: plains zebra ( E. burchelli , with seven subspecies: Damara, E.b. antiquorum ; Burchell’s, E.b. burchellii ; Chapman’s, E.b. chapmannii ; Crawshay’s, E.b. crawshayi ; upper Zambezi, E.b. zambeziensis ; Grant’s, E.b. boehmi ; and the Quagga (extinct), E.b. quagga [54] ). Grevy’s zebra ( E. grevyi ). Mountain zebra ( E. zebra , with two subspecies: Hartman’s, E. z. hartmannae ; and Cape, E. z. zebra ). African wild ass ( E. africanus , with three subspecies: Somali, E. a. somaliensis ; Nubian, E. a. africanus , and Atlas (extinct), E. a. atlanticus ). Przewalski’s horse ( E. ferus przewalksii ). Kiang ( E. kiang , with three subspecies: Eastern, E. k. holdereri ; Western, E. k. kiang ; and southern, E. k. polyodon ). Asiatic wild ass ( E. hemionus , with six subspecies: Mongolian, E. h. hemionus ; Gobi, E. h. leuteus ; Kulan, E. h. kulan ; Onager, E. h. onager ; Indian, E. h. khur ; and Syrian, E. h. hemippus ). Subspecies and species designations were all taken from ref 54 . Mean scores were calculated for each subspecies, and these scores were averaged again to generate species scores. To quantify pelage colouration, we followed the methodology of Groves and Bell [15] and used three of their criteria for each photograph. In brief, they were (a) belly striping, namely, the number of stripes connected to the ventral midline of the animal; (b) shadow stripes: 0=none, 1=poorly developed, 2=clear on rump (the area behind the flank) not on neck, 3=strong on rump and neck; and (c) degree of leg stripes: 0=none, 1=none/traces below elbow and stifle, 2=clearly present to knee/hock, 3=down to hoof, but broken or incomplete, 4=complete, unbroken). In addition, we developed further categories to better capture the variation observed between various zebra subspecies. These were (d) the overall appearance of the colour of the legs (scored as light, medium or dark) from which we created a new measure called leg stripe intensity, namely, the score for leg striping (0–4) multiplied by the colour of the legs (1=white/light, 2=‘black’/dark). This measure, called leg stripe intensity, captures both the degree of striping and the darkness of leg colouration, and ranges from 0 to 8.0. (e) The number of black stripes on the animal’s face, from the end of the solid-coloured portion of the muzzle up to the throat. (f) The number of black stripes from the animal’s throat to the animal’s withers. (g) The number (counted) of vertical body stripes found on the lateral surface (the area between the vertical lines from groin and withers to the elbow) of the animal. This was subsequently recoded into four broad categories to avoid minor differences in stripe number having undue influence: no stripes=0, 1–2.9 stripes=1, 3–6 stripes=2 and >6 stripes=3 and is called flank striping. (h) The number of horizontal stripes (counted) on the rump. This was subsequently recoded into four categories: no stripes=0, 1–4.9 stripes=1, 5–10 stripes=2, and >10 stripes=3 and is called rump striping. We elected to analyse striping patterns on different parts of the body because they varied considerably in width, number and orientation [55] and used a variety of methods including presence, number and intensity of stripes as we do not know to what predators, flies or conspecifics attend. Range maps For the historical ranges of equid subspecies, we used ref. 54 . All species’ range information was taken from this source, except for Przewalski’s horse taken from ref. 56 . Subspecies information on the African wild ass was gleaned from ref. 57 and that on the kiang and Asiatic wild ass was gleaned from ref. 58 . To measure the degree of overlap between equid ranges and our independent variables: predator ranges, temperature ranges, vegetation zones, tsetse fly distributions and proxies for tabanid fly distributions, we used the software ArcGIS 10. We started with a map of the Old World as the basemap (from Natural Earth. Free vector and raster map data; http://www.naturalearthdata.com ) onto which we overlaid the data. Data consisted of range maps for each species or subspecies, and our independent variables that we georeferenced onto the basemap using a minimum of four reference points, and distance errors were minimized to ensure accurate map overlap. Once the range maps were rasterized onto the basemap, polygons were created by ArcGIS; these polygons contain spatial information, such that the size of a particular range as well as the amount of overlap between various polygons can be calculated. We used ArcGIS 10 to determine areas of overlap between each combination of ranges. These areas of overlap were then used to create the percentage overlap of each subspecies’ range with a given independent variable (using R ), and the percent overlaps are used as the data points. To derive accurate overlap information for species distributions, we were careful to select reputable sources for our range information. Information on tsetse fly distribution came from the Food and Agriculture Organization of the United Nations Consultant’s Report, the Predicted Distributions of Tsetse in Africa, published on February 2000 ( http://www.fao.org/ag/againfo/programmes/en/paat/documents/maps/pdf/tserep.pdf ). We used historical presence/absence maps for the superfamily groups, palpalis , morsitans and fusca , which are the standard groups used for tsetse flies. ArcGIS 10 was then able to find the union of these three distributions to determine an overall tsetse distribution in Africa. For presence or absence of predator species, we used historical range information, as geographic ranges of large carnivores have contracted drastically in recent times and historical ranges are most likely to have influenced the evolution of equid colouration. We included the following predators: spotted hyaena ( C. crocuta ), whose historic range was taken from the International Union for Conservation of Nature ( http://www.iucnredlist.org ), lion ( P. leo ), whose historic range was taken from Panthera ( http://www.panthera.org ), tiger ( P. tigris ), whose historic range was taken from Panthera ( http://www.panthera.org ) and wolf ( C. lupus ), whose historic range for Asia was taken from the International Union for Conservation of Nature ( http://www.iucnredlist.org ). All are known to prey on equids. For world vegetation zones, we used a world biome map obtained from http://www.kidsmaps.com/geography/The+World/Economic/Biomes+of+the+World . We chose this source because (i) the website is run by Wikimedia that only contains reviewed sources, (ii) map quality and resolution are high and lean themselves favourably to use in ArcGIS and (iii) the map contains numerous detailed and specific vegetation categories, desirable for our goal of determining whether habitat affects the evolution of animal colouration. Tabanidae comprise over 4,154 species, are found globally except on oceanic islands and at the poles, but only very general distribution maps exist [59] . In temperate zones, they are abundant in summer and in the tropics they principally appear during the wet season. More specifically, optimal tabanid habitat is thought to exist in locations where temperature lies between 15 and 30 °C and humidity is between 30 and 85% (refs 60 , 61 , 62 , 63 , 64 , 65 ). As climate changes from month to month, locations that are in the optimal temperature and humidity range were identified for each month of the year. We used GIS products of maximum daily temperature and daily relative humidity at 15:00 hours, aggregated over each month, generated as output by a recent global climatology effort that aggregates and adjusts historical climate data from across the world [66] . Specifically, we used data on monthly values of humidity and maximum daily temperature that had a resolution of 10 feet squared. We combined the two data files to identify, for each month, which locations were in the optimal range. There is significant intra-annual variation in climate and as such, regions that are optimal for tabanid activity in July are not necessarily optimal in January. Many locations are optimal for a single month, but few are optimal all year round. To identify what effect consistency in optimality has, we identified which locations were frequently optimal and which were rarely optimal. Specifically, we created 12 distinct maps, each one identifying which locations are optimal at least that many months in a row (for example, the fourth map identifies locations that have 4 consecutive months in the optimal range). The first map shows a large range where only one month in the optimal range is needed, while the twelfth map shows the very small range where the temperature and humidity are optimal all year long. All analyses were performed in ArcGIS 10 (to read the initial map files and identify the individual optimal regions) and R 2.15.0 using the programs such as maptools, rgeos and sp (to combine the temperature and humidity maps and construct the 12 distinct maps). All distribution maps of temperature isoclines were obtained from the National Oceanic and Atmospheric Administration ( http://www.noaa.gov ). Mean adult group sizes and maximum herd sizes for each species (but not for subspecies) were taken from the literature ( Supplementary Note 3 ). For a derivation of phylogenies, see Supplementary Note 4 . Phylogenetic analyses As we had many more candidate factors than species or subspecies, we ran single-factor PGLS analyses ( gls function in the ‘nlme’ module [67] with a correlation structure based on the phylogenetic tree) for every explanatory factor (all percent range overlap by tabanid activity (12 versions, 1 through 12 consecutive months), Old World average monthly maximum temperature values reaching 25 °C (and so on for each additional degree up to 30 °C), woodland habitat, tsetse fly range, spotted hyaena range, lion range, mean group size (species level only) and maximum group size (species level only)) against the following quantitative measures of colouration at the species and subspecies level: number of face stripes, number of neck stripes, flank striping, rump striping, shadow stripes, belly stripe number and leg striping intensity. For species-level analyses, given the small number of species ( N =7), we could only test a maximum of four factors simultaneously in one model. We chose the four factors with the lowest P values from the individual PGLS tests and included them in an Akaike Information Criterion correction model selection procedure [68] . To test as many hypotheses as possible, we only allowed one (the lowest P value) tabanid score, one (the lowest P value) temperature score, one predator (hyaena or lion) score, one group size score or one woodland score into these final analyses even if other versions still had lower P values than factors that did enter the model. Using the ‘MuMIn’ module [69] in R, we ran all possible Akaike Information Criterion models including these four factors [68] . Summary statistics from all possible models procedure are presented for each factor weighted by their importance to the best models relative to the worst models [69] . Importance score (I: the sum of the model weights that each factor appears in) ranges from 0 to 1 where 0–0.2=relatively unimportant, 0.2–0.5=moderately important and 0.5–1.0=very important. Procedures were identical for subspecies level tests except that Akaike Information Criterion correction models included six factors: the best tabanid score, the best temperature score, tsetse fly score, hyaena score, lion score and woodland score. For dichotomous colouration scores (presence of stripes (Y/N) at both the species and subspecies level, presence of shadow stripes (Y/N) at the species level), we ran phylogenetically corrected logistic regression models using the compar.gee function in ‘ape.’ We ran single-factor models of all predictor variables similar to the PGLS analyses above and report the results of those individual tests. We reconstructed the evolutionary history of leg stripe intensity using the getAncStates function of the ‘geiger’ module [70] in R. Results of single-factor analyses are the following. Face stripe number. Subspecies level: single-factor analyses (PGLS: N =20) produced P values as follows: maximum temperature of 27 °C ( P =0.6091), 6 consecutive months of tabanid activity ( P =0.0090), tsetse fly distribution ( P =0.7228), woodland ( P =0.4232), hyaena ( P =0.2652) and lion ( P =0.3066). Species level: single-factor analyses (PGLS: N =7) produced P values as follows: maximum temperature of 25 °C ( P =0.2292), 9 consecutive months of tabanid activity ( P =0.0507), tsetse fly distribution ( P =0.0273), woodland ( P =0.5992), hyaena ( P =0.1706), lion ( P =0.1073), mean group size ( P =0.4568) and maximum group size ( P =0.3856). Neck stripe number. Subspecies level: single-factor analyses (PGLS: N =20) produced P values as follows: maximum temperature of 27 °C ( P =0.7739), 6 consecutive months of tabanid activity ( P =0.0404), tsetse fly distribution ( P =0.6089), woodland ( P =0.6773), hyaena ( P =0.5032) and lion ( P =0.3176). Species level: single-factor analyses (PGLS: N =7) produced P values as follows: maximum temperature of 25 °C ( P =0.2527), 9 consecutive months of tabanid activity ( P =0.0531), tsetse fly distribution ( P =0.3410), woodland ( P =0.6024), hyaena ( P =0.1958), lion ( P =0.1092), mean group size ( P =0.4506) and maximum group size ( P =0.3849). Flank striping. Subspecies level: single-factor analyses (PGLS: N =20) produced P values as follows: maximum temperature of 28 °C ( P =0.3379), 8 consecutive months of tabanid activity ( P =0.0148), tsetse fly distribution ( P =0.2843), woodland ( P =0.8234), hyaena ( P =0.0684) and lion ( P =0.4798). Species level: single-factor analyses (PGLS: N =7) produced P values as follows: maximum temperature of 25 °C ( P =0.2534), 8 consecutive months of tabanid activity ( P =0.1259), tsetse fly distribution ( P =0.6370), woodland ( P =0.9686), hyaena ( P =0.1731), lion ( P =0.1327), mean group size ( P =0.4269) and maximum group size ( P =0.4785). Rump striping. Subspecies level: single-factor analyses (PGLS: N =20) produced P values as follows: maximum temperature of 30 °C ( P =0.2697), 9 consecutive months of tabanid activity ( P =0.0107), tsetse fly distribution ( P =0.0098), woodland ( P =0.8657), hyaena ( P =0.0694), lion ( P =0.6576), mean group size ( P =0.4269) and maximum group size ( P =0.4785). Species level: single-factor analyses (PGLS: N =7) produced P values as follows: maximum temperature of 26 °C ( P =0.0752), 7 consecutive months of tabanid activity ( P =0.2106), tsetse fly distribution ( P =0.2168), woodland ( P =0.7545), hyaena ( P =0.0173), lion ( P =0.2294), mean group size ( P =0.6013) and maximum group size ( P =0.6484). Shadow stripe severity. Subspecies level: single-factor analyses (PGLS: N =20) produced P values as follows: maximum temperature of 25 °C ( P =0.7769), 6 consecutive months of tabanid activity ( P =0.0097), tsetse fly distribution ( P =0.5102), woodland ( P =0.7557), hyaena ( P =0.4051) and lion ( P =0.2620). Species level: single-factor phylogenetic logistic regressions ( N =7) at the 0/1 level produced P values as follows: maximum temperature of 25 °C ( P =0.5949), tsetse fly distribution, woodland and 3 up to 11 consecutive months of tabanid activity all showed a perfect fit with the presence of shadow stripes, hyaena ( P =0.5775), lion ( P =0.9099), mean group size ( P =0.9213) and maximum group size ( P =0.6331) but we could not run a multivariate model. Belly stripe number. Subspecies level: single-factor analyses (PGLS: N =20) produced P values as follows: maximum temperature of 26 °C ( P =0.2575), 12 consecutive months of tabanid activity ( P =0.0003), tsetse fly distribution ( P =0.0000), woodland ( P =0.2065), hyaena ( P =0.0323) and lion ( P =0.8798). Species level: single-factor analyses (PGLS: N =7) produced P values as follows: maximum temperature of 30 °C ( P =0.4679), 11 consecutive months of tabanid activity ( P =0.1303), tsetse fly distribution ( P =0.0135), woodland ( P =0.0561), hyaena ( P =0.6573), lion ( P =0.6572), mean group size ( P =0.9683) and maximum group size ( P =0.6045). Leg stripe intensity. Subspecies level: single-factor analyses (PGLS: N =20) produced P values as follows: maximum temperature of 27 °C ( P =0.4226), 7 consecutive months of tabanid activity ( P =0.0010), tsetse fly distribution ( P =0.0309), woodland ( P =0.5981), hyaena ( P =0.0083) and lion ( P =0.3795). Species level: single-factor analyses (PGLS: N =7) produced P values as follows: maximum temperature of 25 °C ( P =0.1200), 7 consecutive months of tabanid activity ( P =0.0514), tsetse fly distribution ( P =0.8803), woodland ( P =0.9094), hyaena ( P =0.0977), lion ( P =0.0312), mean group size ( P =0.1494) and maximum group size ( P =0.2628). We scored hair depths and lengths on museum pelts of equids and artiodactyls that live sympatrically with zebra species ( Supplementary Note 5 ). How to cite this article: Caro, T. et al . The function of zebra stripes. Nat. Commun. 5:3535 doi: 10.1038/ncomms4535 (2014).